Synaptic tagging and capture in the living rat In isolated hippocampal slices, decaying long-term potentiation can be stabilized and converted to late long-term potentiation lasting many hours, by prior or subsequent strong high-frequency tetanization of an independent input to a common population of neurons—a phenomenon known as ‘synaptic tagging and capture’. Here we show that the same phenomenon occurs in the intact rat. Late long-term potentiation can be induced in CA1 during the inhibition of protein synthesis if an independent input is strongly tetanized beforehand. Conversely, declining early long-term potentiation induced by weak tetanization can be converted into lasting late long-term potentiation by subsequent strong tetanization of a separate input. These findings indicate that synaptic tagging and capture is not limited to in vitro preparations; the past and future activity of neurons has a critical role in determining the persistence of synaptic changes in the living animal, thus providing a bridge between cellular studies of protein synthesis-dependent synaptic potentiation and behavioural studies of memory persistence. Throughout the history of neuroscience, discoveries about brain function made in both humans and living animals have triggered research into circuit-level, neuronal and molecular mechanisms. For example, the in vivo discovery of long-term potentiation (LTP) of synaptic strength initiated an explosion of interest in the cellular and molecular mechanisms of synaptic change [1] . Similarly, ocular dominance plasticity was observed almost six decades ago in the cortex of the living cat [2] , triggering computational models [3] and experimental studies in vitro to reveal its physiological basis [4] . The converse is also true; new discoveries at the molecular and cellular level, often in reduced preparations, have led to insights concerning the functioning of the intact nervous system. Examples include classical studies of neuronal plasticity in Aplysia [5] , the in vitro discovery of the homeostatic scaling of synaptic weights [6] , and adult neurogenesis [7] . This interdisciplinary interplay between different levels of analysis is both an exciting feature of contemporary neuroscience and a necessary step towards an integrated functional and mechanistic account of the operation of the brain. Although it is generally naïve to explain complex processes such as vision or memory with reference only to molecular mechanisms, there may be instances in which cellular processes place such rigid constraints on systems-level properties that the gap between levels can be bridged to realize a full understanding. For example, the encoding of memory traces in the mammalian brain requires rapid changes in synaptic efficacy in response to glutamatergic activity, and engages similar cellular mechanisms to those that underlie LTP [1] . If such changes in synaptic strength at a set of synapses cannot be stabilized, it is difficult to imagine how lasting memory traces could be formed [8] . The initial phase of early LTP is supported by the post-translational modification or trafficking of existing proteins, whereas late LTP lasting at least 4–6 h requires new protein synthesis [9] . In vitro studies indicate that the events causing the upregulation of protein synthesis, in the soma or in dendrites, need not occur at exactly the same time as the trigger for LTP induction [10] , [11] , [12] , [13] , [14] , [15] , [16] , [17] , [18] , [19] , [20] , [21] . Two critical observations that underlie the ‘synaptic tagging and capture’ (STC) framework are: (1) late LTP in hippocampal area CA1 can be blocked by protein-synthesis inhibitors such as anisomycin, but prior strong tetanization of an independent input to an overlapping population of postsynaptic neurons stabilizes the decaying LTP [10] —in other words late LTP can be induced without new protein synthesis at the time of induction if the relevant plasticity-related proteins have been synthesized beforehand; and (2) a strong tetanus can also ‘rescue’ decaying LTP induced by subsequent, or prior, weak tetanization of an independent input [10] , [11] , [13] , [14] , [15] , [16] , [17] , [18] , [19] , [21] . This extension of the time window for associative interactions during the stabilization of synaptic changes (sometimes called ‘late associativity’), likely has important implications for our understanding of the association of information across time and the formation of lasting memories. According to the STC hypothesis, glutamatergic stimulation during memory encoding sets temporary ‘tags’ at activated synapses, in a post-translational manner, that then sequester plasticity-related proteins as they become available, thus stabilizing synaptic changes [22] , [23] , [24] . However, the phenomenon of STC has neither been reported nor validated in vivo . Much information has been gathered over the past 10 years concerning the molecular mechanisms underlying the STC process, extending to the level of individual dendritic spines [20] , but it is not yet known whether the level of available proteins places significant restrictions on the persistence of synaptic changes in vivo . Spontaneous activity levels are reduced in vitro , neuromodulatory afferents are severed, and baseline levels of plasticity-related proteins are low if sufficient time is allowed for metabolic stabilization [25] . In the living animal, free from these artificial constraints on protein synthesis, the availability of relevant proteins may not limit the duration of synaptic changes; all synapses that are activated above a certain threshold—and tagged—might successfully capture the proteins necessary for lasting potentiation. In other words, the STC phenomenon might be specific to in vitro preparations, with no relevance in the intact animal. Despite the need for an assessment of synaptic tagging and capture in vivo , the demand for two independent synaptic inputs to a common population of postsynaptic neurons presents a technical challenge [26] . In CA1 slices, two stimulating electrodes can be placed in the Schaffer-collateral pathway, one on either side of a recording electrode in the stratum radiatum, but this configuration does not yield independent inputs in the intact animal. To overcome this difficulty, we chose to exploit the extensive long-range longitudinal connectivity of the Schaffer-collateral/commissural system, in addition to the transverse connectivity that forms part of the ‘traditional’ trisynaptic circuit. The axons of CA3 are extensively collateralized, forming both associational connections with other CA3 cells, as well as the Schaffer-collateral projection to CA1. Axons in both of these projections can extend for distances of several millimetres along the septotemporal (dorso-ventral) axis of the hippocampus; the commissural projection comprises axons that cross the midline via the ventral hippocampal commissure and terminate in the contralateral hippocampus [27] . Functional and anatomical studies indicate that interhippocampal CA3–CA1 connectivity is maximal between regions located at equivalent septotemporal levels, and ipsilateral and contralateral projections converge on an overlapping population of CA1 neurons [28] . By placing stimulating electrodes bilaterally in CA3 at equivalent locations, independent populations of afferents to CA1 can be activated [29] . Using this arrangement, we set out to examine the phenomenon of synaptic tagging and capture in the living animal. In experiment 1, we present evidence that strong tetanization can rescue decaying early LTP induced by subsequent tetanization of a second input in the presence of the protein-synthesis inhibitor anisomycin (‘strong before strong’ [10] ). In experiment 2, we show that early LTP induced by weak tetanization can be stabilized by the later delivery of a strong tetanus to a second input (‘weak before strong’ [11] ). In experiment 3, we investigate the dopamine-dependence of late LTP induced by our strong-tetanus protocol. Overall, our results confirm that ‘synaptic tagging and capture’ can occur in the intact animal, and is not merely an artefact of in vitro hippocampal preparations. Independence of ipsilateral and contralateral projections Bilateral stimulation of CA3 under urethane anaesthesia activated independent ipsilateral (s1 i ) and contralateral (s2 c ) populations of afferents converging on CA1 ( Fig. 1 ). Owing to the challenging nature of the experimental set-up, and the need for long baseline periods to ensure signal stability, the time between the induction of anaesthesia and tetanization was typically 5–6 h, comparable to the incubation periods employed in vitro to minimize background levels of plasticity-related proteins [25] . 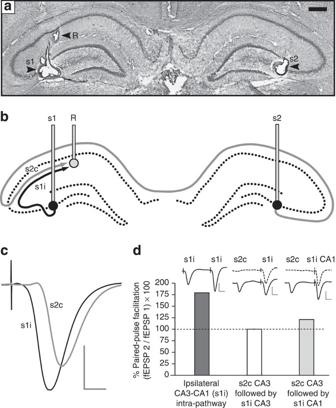Figure 1: Experimental set-up. (a) Photomicrograh of coronal sections indicating the location of bilateral stimulating electrodes in CA3 (s1 and s2) and a recording electrode in left CA1 (R); the right-hand recording electrode was visible only in a slightly more posterior section. Arrows indicate the location of marking lesions made at the electrode tips; scale bar=0.5 mm. (b) Schematic diagram of stimulating and recording sites (s1 and s2), and ipsilateral and contralateral CA3–CA1 projections (s1iand s2c). In this example, both pathways converge on a common population of neurons whose synaptic responses are sampled by the left-hand recording electrode, R. For simplicity, CA3–CA3 projections are omitted (seeSupplementary Methods). (c) Representative fEPSPs evoked by stimulation of s1iand s2c. Note the longer latency and smaller amplitude of the contralateral fEPSP (scale bar: vertical=2 mV; horizontal=5 ms). (d) Intra-pathway paired stimulation at an interval of 50 ms yielded pronounced PPF of the fEPSP slope; the left-hand bar shows a single example of PPF in the ipsilateral CA3–CA1 projection; examples of fEPSPs elicited by paired stimulation are shown. However, PPF was absent after stimulation of s2cfollowed by s1iat an interval of 50 ms; the middle bar shows mean (±s.e.m.) PPF for all experiments reported inFigs 2and4(n=51), a value that did not differ from chance (100%) (100.2±0.8;t(50)=0.20;P>0.8; one-samplet-test), confirming the independence of the two pathways. Independence was compromised if one or both stimulating electrodes were raised into CA1; the right-hand bar shows an example of modest PPF obtained in a single rat by paired stimulation of contralateral CA3 followed by ipsilateral CA1, indicating that the two stimulators now activate partially overlapping populations of afferents. Examples of fEPSPs elicited by stimulation of s1iwith (solid line) or without (dashed line) prior stimulation of s2care shown above the middle and right-hand bars (scale bar: vertical=4 mV; horizontal=10 ms). Figure 1: Experimental set-up. ( a ) Photomicrograh of coronal sections indicating the location of bilateral stimulating electrodes in CA3 (s1 and s2) and a recording electrode in left CA1 (R); the right-hand recording electrode was visible only in a slightly more posterior section. Arrows indicate the location of marking lesions made at the electrode tips; scale bar=0.5 mm. ( b ) Schematic diagram of stimulating and recording sites (s1 and s2), and ipsilateral and contralateral CA3–CA1 projections (s1 i and s2 c ). In this example, both pathways converge on a common population of neurons whose synaptic responses are sampled by the left-hand recording electrode, R. For simplicity, CA3–CA3 projections are omitted (see Supplementary Methods ). ( c ) Representative fEPSPs evoked by stimulation of s1 i and s2 c . Note the longer latency and smaller amplitude of the contralateral fEPSP (scale bar: vertical=2 mV; horizontal=5 ms). ( d ) Intra-pathway paired stimulation at an interval of 50 ms yielded pronounced PPF of the fEPSP slope; the left-hand bar shows a single example of PPF in the ipsilateral CA3–CA1 projection; examples of fEPSPs elicited by paired stimulation are shown. However, PPF was absent after stimulation of s2 c followed by s1 i at an interval of 50 ms; the middle bar shows mean (±s.e.m.) PPF for all experiments reported in Figs 2 and 4 ( n =51), a value that did not differ from chance (100%) (100.2±0.8; t (50)=0.20; P >0.8; one-sample t -test), confirming the independence of the two pathways. Independence was compromised if one or both stimulating electrodes were raised into CA1; the right-hand bar shows an example of modest PPF obtained in a single rat by paired stimulation of contralateral CA3 followed by ipsilateral CA1, indicating that the two stimulators now activate partially overlapping populations of afferents. Examples of fEPSPs elicited by stimulation of s1 i with (solid line) or without (dashed line) prior stimulation of s2 c are shown above the middle and right-hand bars (scale bar: vertical=4 mV; horizontal=10 ms). Full size image ‘Strong-before-strong’ protocol Experiment 1 involved strong tetanization of pathway s1 i after artificial cerebrospinal fluid (aCSF) infusion (‘strong+aCSF’ group; n =6), which induced persistent LTP lasting at least 5 h, relative to a non-tetanized contralateral control pathway (s2 c ) ( Fig. 2a and d ). Intraventricular infusion of anisomycin (ANI) before strong tetanization of s1 i (‘strong+ANI’ group; n =7) spared post-tetanic potentiation (PTP), and the early phase of LTP, but late LTP was completely blocked; potentiation lasted ~3 h relative to the control pathway ( Fig. 2b and d ). Strong tetanization of s2 c before anisomycin infusion and subsequent tetanization of s1 i (‘strong-before-strong+ANI’ group) yielded late LTP not only in s2 c , but also in s1 i , despite the fact that LTP in s1 i was induced during the inhibition of protein synthesis ( Fig. 2c and d ). These results indicate that the persistence of LTP is dissociable from its initial strength, consistent with the STC hypothesis. An analysis of the opposite, mirror-image situation—the rescue of LTP in the contralateral projection (s1 c ) by strong tetanization of the ipsilateral pathway (s2 i ) in the same animals—is presented in Supplementary Figs S1 and S2 , and Supplementary Table S1 . 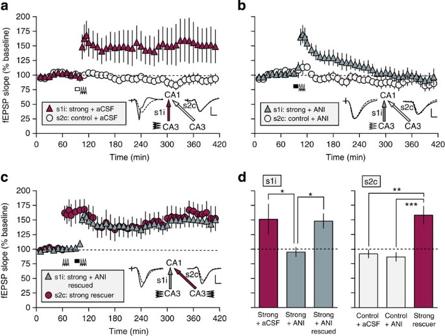Figure 2: Strong-before-strong protocol. (a) Bilateral intraventricular infusion of aCSF (white rectangle) starting 15 min before strong tetanization of s1i(arrowheads) had no effect on late LTP in s1i(‘strong+aCSF’;n=6). (b) Infusion of anisomycin (black rectangle) completely blocked late LTP in s1i(‘strong+ANI’;n=7). (c) The addition of a strong tetanus to s2cending 15 min before the start of anisomycin infusion and tetanization of s1iresulted in late LTP in both pathways (‘strong-before-strong+ANI’ group, comprising ‘strong+ANI rescued’ and ‘strong rescuer’ pathways;n=9). Sample fEPSPs recorded in s1iand s2cbefore (dotted line) and 5 h after tetanization (solid line) are shown (scale bars for a-c: vertical=2 mV; horizontal=5 ms). (d) Mean fEPSP slope values recorded for s1iand s2cin all experimental groups between 4–5 h after the relevant tetanus, and normalized to the mean of the 1-h baseline period. Asterisks indicate significant group differences in late LTP (*P<0.05; **P<0.01; ***P<0.001;post-hoccomparisons—Fisher’s LSD). All data are plotted as mean±s.e.m. Figure 2: Strong-before-strong protocol. ( a ) Bilateral intraventricular infusion of aCSF (white rectangle) starting 15 min before strong tetanization of s1 i (arrowheads) had no effect on late LTP in s1 i (‘strong+aCSF’; n =6). ( b ) Infusion of anisomycin (black rectangle) completely blocked late LTP in s1 i (‘strong+ANI’; n =7). ( c ) The addition of a strong tetanus to s2 c ending 15 min before the start of anisomycin infusion and tetanization of s1 i resulted in late LTP in both pathways (‘strong-before-strong+ANI’ group, comprising ‘strong+ANI rescued’ and ‘strong rescuer’ pathways; n =9). Sample fEPSPs recorded in s1 i and s2 c before (dotted line) and 5 h after tetanization (solid line) are shown (scale bars for a-c: vertical=2 mV; horizontal=5 ms). ( d ) Mean fEPSP slope values recorded for s1 i and s2 c in all experimental groups between 4–5 h after the relevant tetanus, and normalized to the mean of the 1-h baseline period. Asterisks indicate significant group differences in late LTP (* P <0.05; ** P <0.01; *** P <0.001; post-hoc comparisons—Fisher’s LSD). All data are plotted as mean±s.e.m. Full size image An analysis of variance (ANOVA) of the percentage field excitatory postsynaptic potential (fEPSP) slope LTP 4–5 h after tetanization ( Fig. 2d ), with group (‘strong+aCSF’, ‘strong+ANI’, and ‘strong before strong+ANI’) as a between-subjects factor, and pathway (s1 i and s2 c ) as a within-subjects factor, revealed a group x pathway interaction (F(2,19)=4.81; P <0.02; Fig. 2d ). Following the overall ANOVA, a separate ANOVA of late LTP in s1 i only revealed a main effect of group (F(2,19)=3.86; P <0.05; Fig. 2d ; left-hand panel). Post-hoc comparisons (Fisher’s LSD) revealed that anisomycin resulted in significantly lower late LTP relative to that in aCSF-treated controls ( P <0.02), but prior tetanization of s2 c resulted in a significant increase in late LTP in s1 i following anisomycin infusion ( P <0.05); the resulting level of LTP did not differ from that in the aCSF-treated group ( P >0.5); and was significantly above baseline (t(8)=3.94; P <0.005; one-sample t -test). Analysis of simple main effects based on the overall ANOVA revealed significant differences between s1 i and s2 c in the ‘strong+aCSF’ group ( P <0.005), indicating significant late LTP, but no difference was observed in the ‘strong+ANI’ group ( P >0.6)—LTP had decayed to baseline values in this case. A main effect of group was also observed in s2 c alone (F(2,19)=12.4; P <0.001; Fig. 2d ; right-hand panel). Post-hoc comparisons (Fisher’s LSD) revealed that a strong tetanus to s2 c in the ‘strong-before-strong+ANI’ group caused significant late LTP relative to the aCSF control pathway ( P <0.001), and the anisomycin control pathway ( P <0.0005); these control pathways did not differ from each other ( P >0.6). At the dose used, anisomycin infusion typically caused a small but rapid increase in the fEPSP, followed by a gradual, but again slight, fall evident in the untetanized control pathway ( Fig. 2b ). However, control pathways did not differ significantly between aCSF- and anisomycin-treated groups 5 h after tetanization (see above), indicating that the block of late LTP cannot be attributed to baseline effects. Group differences in PTP (the mean slope during the 5-min period after the final tetanus train) and early LTP (30–60 min after the final tetanus train) did not reach significance (F<1 in both cases; ANOVA), indicating that anisomycin predominantly impaired late LTP. Nonetheless, higher doses caused pronounced baseline changes ( Fig. 3 ). 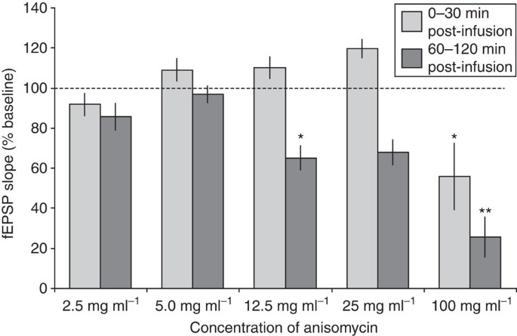Figure 3: Dose-dependent depression of the fEPSP slope by higher doses of anisomycin. fEPSP slope 0–30 and 60–120 min after the end of drug infusion (as a percentage of the value recorded during a 30-min baseline period) is plotted for a range of doses of anisomycin (expressed as μg μl−1). All doses were delivered in a total volume of 10 μl (5 μl per ventricle) over 10 min. As the effects of anisomycin were proportionally similar in both ipsilateral and contralateral CA3–CA1 pathways, data from all pathways were combined in this analysis (2.5 μg μl−1:n=6 (3 rats); 5.0 μg μl−1:n=13 (8 rats; data from all control pathways in ‘ANI+strong’ group,Fig. 2); 12.5 μg μl−1:n=4 (1 rat); 25 μg μl−1:n=4 (1 rat); 100 μg μl−1:n=8 (2 rats)). A main effect of dose was observed both 0–30 min (F(4,30)=6.15;P<0.002) and 60–120 min post-infusion (F(4,30)=19.3;P<0.001). Asterisks indicate significant deviations from baseline (100%; **P<0.01; *P<0.05; one-samplet-tests with Bonferroni correction). All data are plotted as mean±s.e.m. Figure 3: Dose-dependent depression of the fEPSP slope by higher doses of anisomycin. fEPSP slope 0–30 and 60–120 min after the end of drug infusion (as a percentage of the value recorded during a 30-min baseline period) is plotted for a range of doses of anisomycin (expressed as μg μl −1 ). All doses were delivered in a total volume of 10 μl (5 μl per ventricle) over 10 min. As the effects of anisomycin were proportionally similar in both ipsilateral and contralateral CA3–CA1 pathways, data from all pathways were combined in this analysis (2.5 μg μl −1 : n =6 (3 rats); 5.0 μg μl −1 : n =13 (8 rats; data from all control pathways in ‘ANI+strong’ group, Fig. 2 ); 12.5 μg μl −1 : n =4 (1 rat); 25 μg μl −1 : n =4 (1 rat); 100 μg μl −1 : n =8 (2 rats)). A main effect of dose was observed both 0–30 min (F(4,30)=6.15; P <0.002) and 60–120 min post-infusion (F(4,30)=19.3; P <0.001). Asterisks indicate significant deviations from baseline (100%; ** P <0.01; * P <0.05; one-sample t -tests with Bonferroni correction). All data are plotted as mean±s.e.m. Full size image To assess the stability of rescued LTP, independently of its magnitude [18] , we carried out an ANOVA of the percentage fEPSP slope LTP 30–60 min and 4–5 h after tetanization in the s1 i pathways of the ‘strong+ANI’ ( Fig. 2b ), and ‘strong-before-strong+ANI’ ( Fig. 2c ) groups only. This analysis revealed a significant group x time interaction (F(1,14)=10.0; P <0.001), and a subsequent analysis of simple main effects revealed a significant decay of LTP between time points in the ‘strong+ANI’ group (F(1,14)=27.7; P <0.001), but no significant decline in the ‘strong-before-strong+ANI’ group (F(1,14)=1.41; P >0.2), confirming the stability of rescued late LTP. There were no group differences in stimulation intensity (F<1; ANOVA) or fEPSP slope over the 1-h baseline period (F(2,19)=1.03; P >0.3); fEPSP slopes in s2 c were significantly smaller than in s1 i (F(1,19)=17.9; P <0.0005), but stimulation intensity did not differ between pathways (F<1). Overall, no significant paired-pulse facilitation (PPF) was observed (t(21)=0.04; P >0.9; one-sample t -test; comparison with chance=100%), and no group differences in values were obtained (F<1). See Table 1 for details. Table 1 Baseline parameters. Full size table ‘Weak-before-strong’ protocol Experiment 2 avoided the use of drugs. Strong tetanization of s1 i (‘strong-only’ group; n =7) induced robust late LTP ( Fig. 4a and d ), whereas weak tetanization (‘weak-only’ group; n =11) induced only a decaying early LTP lasting ~3 h relative to the untetanized control pathway (s2 c ) ( Fig. 4b and d ). However, strong tetanization of s2 c after weak tetanization of s1 i (‘weak-before-strong’ group; n =11) not only induced late LTP in s2 c , but also rescued late LTP in s1 i ( Fig. 4c and d ). In other words, decaying potentiation induced by weak tetanization can be converted into late LTP by strong tetanization delivered later to an independent input. An analysis of the opposite, mirror-image situation—the rescue of LTP in the contralateral projection (s1 c ) by strong tetanization of the ipsilateral pathway (s2 i )—is presented in Supplementary Figs S1 and S3 and Supplementary Table S1 . 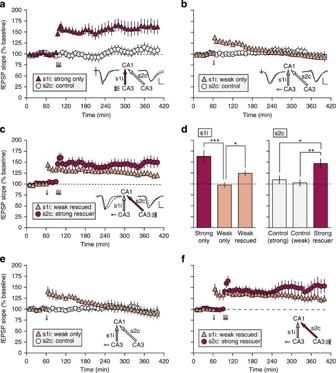Figure 4: Weak-before-strong protocol. (a) Strong tetanization (arrowheads) of ipsilateral CA3 (s1i) induced stable late LTP (‘strong only’;n=7). (b) Weak tetanization of s1i(arrowhead) induced decremental early LTP that reached baseline within ~3 h (‘weak only’;n=11). (c) Strong tetanization of s2c30 min after weak tetanization of s1iresulted in late LTP in both pathways (‘weak before strong’;n=11). Sample fEPSPs recorded in s1iand s2cbefore (dotted line) and 5 h after tetanization (solid line) are shown ina–c(scale bar: vertical=2 mV; horizontal=5 ms). (d) Mean normalized fEPSP slope in s1iand s2crecorded 4–5 h after tetanization in all groups. Asterisks indicate significant differences in late LTP between groups (*P<0.05; **P<0.01; ***P<0.001;post-hoccomparisons—Fisher’s LSD). (e,f) Re-analysis of ‘weak-only’ (e;n=8) and ‘weak-before-strong’ (f;n=7) data after the exclusion of data from all animals in which baseline fEPSP slope values fell by >10 percentage points between the first and last 20-min periods of the 1-h baseline in either s1ior s2c. The pattern of results is identical to that observed in (b) and (c). All data are plotted as mean±s.e.m. Figure 4: Weak-before-strong protocol. ( a ) Strong tetanization (arrowheads) of ipsilateral CA3 (s1 i ) induced stable late LTP (‘strong only’; n =7). ( b ) Weak tetanization of s1 i (arrowhead) induced decremental early LTP that reached baseline within ~3 h (‘weak only’; n =11). ( c ) Strong tetanization of s2 c 30 min after weak tetanization of s1 i resulted in late LTP in both pathways (‘weak before strong’; n =11). Sample fEPSPs recorded in s1 i and s2 c before (dotted line) and 5 h after tetanization (solid line) are shown in a – c (scale bar: vertical=2 mV; horizontal=5 ms). ( d ) Mean normalized fEPSP slope in s1 i and s2 c recorded 4–5 h after tetanization in all groups. Asterisks indicate significant differences in late LTP between groups (* P <0.05; ** P <0.01; *** P <0.001; post-hoc comparisons—Fisher’s LSD). ( e , f ) Re-analysis of ‘weak-only’ ( e ; n =8) and ‘weak-before-strong’ ( f ; n =7) data after the exclusion of data from all animals in which baseline fEPSP slope values fell by >10 percentage points between the first and last 20-min periods of the 1-h baseline in either s1 i or s2 c . The pattern of results is identical to that observed in ( b ) and ( c ). All data are plotted as mean±s.e.m. Full size image An ANOVA of the mean percentage fEPSP slope LTP 4–5 h after tetanization, with group (‘weak only’, ‘strong only’ and ‘weak before strong’) as a between-subjects factor, and pathway (s1 i and s2 c ) as a within-subjects factor, revealed a group x pathway interaction (F(2,26)=9.35; P <0.002; Fig. 4d ). Following the overall ANOVA, a separate ANOVA of late LTP in s1 i only revealed a main effect of group (F(2,26)=11.9; P <0.0005; Fig. 4d ; left-hand panel). Post-hoc comparisons (Fisher’s LSD) revealed that a weak tetanus to s1 i caused significantly less late LTP than a strong tetanus to s1 i ( P <0.0005), but pathway s1 i in the ‘weak-before-strong’ group showed significantly more late LTP than the same pathway in the weak-only group ( P <0.05)—in other words a rescue of LTP was observed. Although the level of late LTP in pathway s1 i of the ‘weak-before-strong’ group remained below that observed in the ‘strong-only’ group ( P <0.001), it was stable and the rescued LTP remained significantly above baseline 4–5 h after tetanization (t(10)=3.59; P <0.005; one-sample t -test). Analysis of simple main effects based on the overall ANOVA revealed significant differences between pathways s1 i and s2 c in the ‘strong-only’ group ( P <0.002), indicating significant late LTP, but no difference was observed in the weakly tetanized group ( P >0.6)—LTP had decayed to baseline values in these animals. A separate analysis of LTP 5–6 h after tetanization gave similar results ( Supplementary Fig. S4 ). A main effect of group was also observed in s2 c alone (F(2,26)=6.21; P <0.01; Fig. 4d , right-hand panel). Post-hoc comparisons (Fisher’s LSD) revealed that a strong tetanus to s2 c in the ‘weak-before-strong’ group caused significant L-LTP relative to the ‘strong-only’ control pathway ( P <0.02), and the ‘weak-only’ control pathway ( P <0.005); these control pathways did not differ from each other ( P >0.6). Owing to the slightly smaller PTP induced by weak (versus strong) tetanization, there was a trend towards a significant overall group difference in PTP in s1 i (F(2,26)=3.20; 0.1> P >0.05; ANOVA). Similarly, an overall analysis of early LTP (30–60 min after tetanization) revealed a significant group effect owing to the inclusion of the ‘strong-only’ group (F(2,26)=5.46; P <0.02). Nevertheless, early LTP did not differ between ‘weak-only’ and ‘weak-before-strong’ groups ( P <0.05; Fisher’s LSD), indicating that late, but not early LTP was significantly facilitated by the strong ‘rescue’ tetanus. As in experiment 1, to assess the stability of rescued LTP induced by a weak tetanus, we conducted an ANOVA of the percentage fEPSP slope LTP 30–60 min and 4–5 h after tetanization in the s1 i pathways of the ‘weak-only’ ( Fig. 4b ), and ‘weak-before-strong’ ( Fig. 4c ) groups only. This analysis revealed a significant group x time interaction (F(1,20)=7.14; P <0.02), and a subsequent analysis of simple main effects revealed a significant decay of LTP between time points in the ‘weak-only’ group (F(1,20)=30.4; P <0.001), but no significant decline in the ‘weak-before-strong’ group (F(1,20)=2.96; P >0.1). There were no group differences in stimulation intensity or fEPSP slope over the 1-h baseline period (F<1 in both cases; ANOVA); fEPSP slopes in s2 c were significantly smaller than in s1 i (F(1,26)=44.7; P <0.0005), but stimulation intensity did not differ between pathways (F<1). Overall, no significant PPF was observed (t(28)=0.29; P >0.7; one-sample t -test; comparison to chance=100%), and no group differences in values were obtained (F<1). See Table 1 . Owing to the slight baseline rise evident in Fig. 4c , data from ‘weak-only’ and ‘weak-before-strong’ groups were re-analysed after the exclusion of data from all animals in which baseline fEPSP slope values rose or fell by more than 10 percentage points between the first and last 20-min periods of the 1-h baseline in either s1 i or s2 c (an analysis that was possible owing to the relatively large n of 11 in these two groups originally). The re-analysed data are shown in Fig. 4e and f (‘weak only’: n =8; ‘weak before strong’: n =7). As expected, baseline values are stable, and the results are numerically very similar to those in Fig. 4b and c . An ANOVA of the mean percentage fEPSP slope LTP 4–5 h after tetanization—with pathway as a within-subjects factor and group as a between-subjects factor—revealed a significant overall main effect of group (F(1,13)=12.8; P <0.005). Comparison of late LTP in pathway s1 i of the ‘weak-only’ and ‘weak-before-strong’ groups revealed a significant difference (F(1,13)=6.52; P <0.025; analysis of simple main effects); late LTP in the latter group remained significantly above chance (t(6)=2.78; P <0.05; one-sample t -test). As expected, the strong rescue tetanus resulted in significant potentiation relative to the untetanized control in the ‘weak-only’ group (F(1,13)=7.92; P <0.02; analysis of simple main effects). The role of dopamine In experiment 3, we assessed the impact of the dopamine antagonist SCH23390 on late LTP. Neither aCSF ( Fig. 5a ; n =7) nor SCH23390 (5 μg μl −1 ; Fig. 5b ; n =7) blocked potentiation after 4 h (the point at which recording ended in this experiment), although a modest fall in both tetanized and control pathways was evident in the SCH23390 group by the end of the recording period. An ANOVA of LTP 3–4 h after tetanization revealed a difference between tetanized and non-tetanized pathways (F(1,12)=13.16; P <0.005), but no effect of drug group (F(1,12)=0.63; P >0.4), and no group × pathway interaction (F(1,12)=0.03; P >0.8). Similarly, no group differences in PTP (0–5 min after tetanus) or early LTP (30–60 min after tetanus) were observed in s1 i (F<1 in both cases). Fig. 5c shows the normalized fEPSP slope in each tetanized pathway expressed as a percentage of the value recorded in the corresponding control pathway, in order to control for baseline changes. When analysed in this way, the time course and level of potentiation were identical in SCH23390 and vehicle-treated groups. Mean potentiation 3-4 h after tetanization is summarized in Fig. 5d . 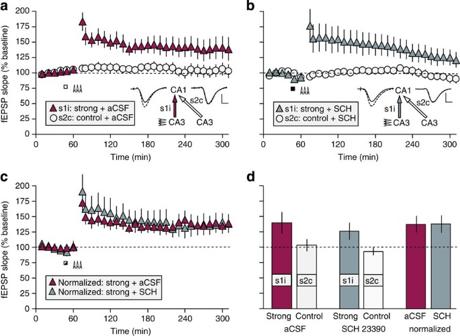Figure 5: Dopamine and late LTP. (a) Bilateral intraventricular infusion of aCSF (n=7; white rectangle) starting 15 min before strong tetanization of s1i(arrowheads) had no effect on late LTP in s1i. (b) Despite a slight baseline fall in both s1iand s2cafter infusion, SCH23390 (n=7; black rectangle) likewise failed to block late LTP. Sample fEPSPs recorded in s1iand s2cbefore (solid line) and 4 h after tetanization (dotted line) are shown inaandb(scale bar: vertical=2 mV; horizontal=5 ms). (c) To eliminate the possible influence of infusion-related baseline changes, values in s1iwere normalized, in each animal, to those in s2cand the mean data were re-plotted (see Methods). SCH23390 had no effect on normalized levels of LTP. The point of drug infusion is indicated by a black-and-white rectangle. (d) Mean normalized fEPSP slope recorded 3-4 h after tetanization in all groups. All data are plotted as mean±s.e.m. Figure 5: Dopamine and late LTP. ( a ) Bilateral intraventricular infusion of aCSF ( n =7; white rectangle) starting 15 min before strong tetanization of s1 i (arrowheads) had no effect on late LTP in s1 i . ( b ) Despite a slight baseline fall in both s1 i and s2 c after infusion, SCH23390 ( n =7; black rectangle) likewise failed to block late LTP. Sample fEPSPs recorded in s1 i and s2 c before (solid line) and 4 h after tetanization (dotted line) are shown in a and b (scale bar: vertical=2 mV; horizontal=5 ms). ( c ) To eliminate the possible influence of infusion-related baseline changes, values in s1 i were normalized, in each animal, to those in s2 c and the mean data were re-plotted (see Methods). SCH23390 had no effect on normalized levels of LTP. The point of drug infusion is indicated by a black-and-white rectangle. ( d ) Mean normalized fEPSP slope recorded 3-4 h after tetanization in all groups. All data are plotted as mean±s.e.m. Full size image No significant group (F(1,12)=0.08; P >0.7) or pathway (F(1,12)=2.07; P >0.1) differences were found in stimulation intensity; baseline fEPSP slope likewise did not differ between groups (F(1,12=0.18; P >0.6), and on this occasion no differences were found between pathways s1 i and s2 c (F(1,12)=1.28; P >0.2); see Table 1 . The results of experiment 1 reveal that late LTP of the ipsilateral Schaffer-collateral input to CA1 (s1 i ) can be induced in the living rat during the inhibition of protein synthesis—a treatment that otherwise limits the duration of LTP to around 3 h—provided that strong tetanization of an independent contralateral commissural input (s2 c ) occurs beforehand ( Fig. 2 ). This suggests that proteins synthesized following strong tetanization of one pathway can subsequently be captured by tags set at the synapses of a separate input. Doses of anisomycin comparable to that used here have previously been reported to block hippocampal LTP, long-term memory formation, and tetanus-induced protein synthesis [30] , [31] , [32] . A large number of proteins are upregulated following the induction of late LTP (for example, McNair et al . [33] ), and there is mounting evidence for the importance of local dendritic translation (for example, refs 34 , 35 , 36 , 37 ). Although we cannot rule out the possibility that anisomycin also blocks long-lasting changes in the intrinsic properties of neurons induced by strong tetanization [38] , a cell-wide mechanism cannot explain the ‘weak-before-strong’ data of experiment 2 (see below), unless weak tetanization sets a synaptic tag as our hypothesis indicates that it must. In our hands, higher doses of anisomycin caused dose-dependent changes in baseline fEPSPs even in the absence of tetanization ( Fig. 3 ), consistent with the multiple effects of anisomycin reported at doses higher than that used in the present study [32] , [39] , [40] , [41] , including the suppression of neural activity [42] . However, no significant baseline changes were observed at the dose used in experiment 1. Experiment 2 reveals that decaying early LTP induced by weak tetanization of the ipsilateral CA3–CA1 projection (s1 i ) can be converted into late LTP by strong tetanization delivered later to the contralateral pathway (s2 c ) ( Fig. 4 ). The delivery of the strong ‘rescue’ tetanus after the weak tetanus excludes the possibility of sensitization, or a reduction in the threshold for the induction of late LTP [11] ; it is consistent with the setting of synaptic tags that subsequently capture proteins synthesized after the strong tetanus, and implies that the availability of plasticity-related proteins can indeed determine the duration of synaptic changes in vivo . Taken together, our results confirm the symmetrical nature of the synaptic tagging and capture process as characterized in vitro —strong tetanization can rescue decaying potentiation whether delivered before or after the latter’s induction [10] , [11] . Although we have focussed on the rescue of LTP in the uncrossed CA3–CA1 projection (s1 i ) by strong tetanization of the crossed pathway (s2 c ), the ability of strong ipsilateral CA3–CA1 tetanization to rescue decaying LTP in the contralateral projection was qualitatively similar, although statistically less robust ( Supplementary Figs S2 and S3 ), perhaps owing to the typically smaller and more variable levels of LTP seen in the crossed CA3–CA1 pathway [43] . In order to obtain independent synaptic inputs to a common pool of CA1 neurons, we stimulated bilaterally in CA3; our electrode locations yielded large fEPSPs in CA1 stratum radiatum following both ipsilateral and contralateral stimulation. The independence of crossed and uncrossed projections was confirmed by the absence of PPF following alternate stimulation of each pathway at an interval of 50 ms ( Fig. 1d , middle bar); similarly, tetanization of one pathway caused no change in the other input. Although commissural projections to CA1 typically exhibit a denser pattern of termination in stratum oriens, relative to ipsilateral inputs that primarily target stratum radiatum, afferents originating from the intrahilar region are predominantly directed toward the contralateral stratum radiatum [44] . In view of this, the recording of large contralateral CA3–CA1 fEPSPs in stratum radiatum is consistent with our placement of stimulating electrodes towards the proximal (dentate) end of CA3. Although our experiments were conducted under urethane—an anaesthetic that suppresses fEPSPs, and necessitates the use of stronger tetanization protocols for LTP induction [45] —strong tetanization induced persistent LTP that was blocked by anisomycin ( Fig. 2b ), suggesting that protein synthesis-dependent late LTP can still be induced under these circumstances. Late LTP typically lasted as long as stable recordings could be maintained (that is, at least 5 h); in some instances, we observed stable LTP for over 10 h following strong tetanization. Having established that synaptic tagging and capture can occur in vivo , it is necessary to identify physiologically plausible neural analogues of the strong tetanus—that is, triggers for the heterosynaptic stabilization of synaptic potentiation induced by the activation of glutamate receptors. As the activation of dopaminergic afferents is a leading candidate for this role [46] , [47] , the absence of an effect of dopamine receptor blockade on LTP induced by the strong tetanus used in the current series of experiments ( Fig. 5 ) might seem surprising. The route of administration and dosage were chosen to match exactly those used in a previous behavioural study in which SCH23390 caused a marked impairment of long-term spatial-memory formation [48] . Moreover, dopamine D1/D5 receptor blockade can block CA1 late LTP in vivo [49] , [50] , and dopamine receptor activation can induce dendritic protein synthesis [51] . But despite the frequent focus on the dopaminergic innervation of CA1, there are likely to be multiple determinants of protein availability. For example, β-adrenergic activation facilitates a form of LTP requiring dendritic translation but not transcription [52] , and somatic action potentials induced by alvear stimulation are sufficient to convert early to late LTP in CA1 (ref. 13 ). In our experiments, it is likely that strong glutamatergic stimulation was sufficient to induce late LTP without the additional requirement for dopaminergic activity; the activation of CaMKIV or metabotropic glutamate receptors might, for example, serve this function [18] , [53] . In fact, for anatomical reasons, the finding that our strong tetanus induces dopamine-independent LTP is fully consistent with the results obtained. The hippocampus receives dopaminergic inputs from mesolimbic structures such as the ventral tegmental area; afferents terminate in CA1 and to a lesser extent in CA3 (ref. 54 ). However, the axons of dopaminergic neurons exhibit limited collateralization, and only around 10% of ventral tegmental area dopaminergic neurons project contralaterally [54] . For these reasons, it is unlikely that tetanization of CA3 could result in a significant recruitment of dopaminergic fibres terminating contralaterally in CA1. In other words, the ability of a strong tetanus delivered to the crossed CA3–CA1 pathway to rescue decaying LTP in the ipsilateral projection is unlikely to be mediated by dopaminergic afferents. Nonetheless, dopamine is likely to have an important role in the stabilization of learning-induced synaptic changes triggered by physiological patterns of stimulation [48] , [55] , [56] . In summary, we find that the synaptic tagging and capture phenomenon, consistent with its hypothesized role in memory [57] , [58] , [55] , is not limited to in vitro preparations. As well as providing a mechanism for the association of information over time, our use of long-range commissural projections to provide the ‘rescue’ stimulus indicates that the information to be associated can originate from cells located in opposite hemispheres of the brain. In other words, the ‘late associativity’ of LTP operates not only over an extended time-frame, but also over a distance of several millimetres in the living rat. Our findings provide a bridge between investigations of behavioural tagging in freely moving animals and in vitro studies of underlying mechanisms, and so validate further work aimed at uncovering the molecular basis of memory persistence. Subjects All procedures were conducted in accordance with the UK Animals (Scientific Procedures) Act (1986). Before the experiment, adult male Lister-hooded rats (250–500 g; n =91) were given ad libitum access to food and water and maintained on a 12-h light/12-h dark cycle. Anaesthesia Rats were anaesthetized with urethane (ethyl carbamate; 1.5 g kg −1 ; 0.3 mg ml −1 , i.p. ), injected with carprofen (Rimadyl small animal solution, 4 mg kg −1 ; s.c.), and placed in a stereotaxic frame with the skull horizontal. Body temperature was monitored by a rectal probe and maintained at 36.2 °C using an isothermic heating blanket. Depth of anaesthesia was assessed throughout the experiment, and urethane top-ups of 0.2 ml were administered as required. Breathing rate was monitored continuously using a light-dependent resistor to detect thoracic movements, and analysed online using in-house software. If breathing fell below 70 breaths per min, rats received an injection of atropine (0.4 mg kg −1 ; s.c.) or doxapram (5 mg kg −1 ; i.p.). Subcutaneous injections of a glucose/saline mixture were administered every 3 h to maintain hydration (1.5 ml of 0.9% saline+0.5 ml of 5% glucose). Electrophysiological recording PTFE-insulated monopolar platinum/iridium recording electrodes (diameter=0.103 mm) were lowered bilaterally into the stratum radiatum of area CA1 (3.8 mm posterior and 2.5 mm lateral to bregma; depth ~−2.5 mm from dura). Bipolar stimulating electrodes comprising two twisted wires identical in composition to the recording electrodes were lowered bilaterally into CA3 (3.5 mm posterior and 3.0 mm lateral to bregma; depth ~−3.0 mm from dura) in order to activate independent populations of synaptic contacts made by ipsilateral Schaffer-collateral (s1 i ) and contralateral commissural projections (s2 c ) converging on the same neuronal populations sampled by each of the recording electrodes. Fig. 1a shows a photomicrograph of representative marking lesions made at both stimulating sites and the left-hand recording site in an individual rat. A schematic illustration of the electrode locations and pathways stimulated is shown Fig. 1b ; for simplicity, CA3–CA3 projections are omitted, and only a single pair of ipsilateral and contralateral projections is shown; in practice CA3 stimulation simultaneously activates crossed and uncrossed afferents, and recording electrodes were placed bilaterally to capitalize on this ( Supplementary Fig. S1 ). Nonetheless; in our main analysis ( Figs 2 and 4 ), we focus solely on the rescue of LTP in an ipsilateral CA3–CA1 projection (s1 i ) by strong tetanization of the crossed CA3–CA1 pathway (s2 c ) converging on the same recording site. Note that the hemisphere (left or right) containing the ipsilateral projection of interest (s1 i ) was varied over days in a quasi-random fashion. An analysis of the opposite, mirror-image situation—the rescue of LTP in the contralateral projection (s1 c ) by strong tetanization of the ipsilateral pathway (s2 i ) in the same animals—is presented in the Supplementary Information ( Supplementary Figs S2 and S3 ). Throughout the experiment, fEPSPs were amplified and sampled at 20 kHz using a PC running custom-written LabView software developed by Patrick Spooner; fEPSP amplitude and initial slope (measured by linear regression between two fixed time points) were monitored on-line. Stimulation was delivered under computer control via a Neurolog system (NL800A; Digitimer LTD, Herts., UK), and consisted of biphasic constant-current pulses. At the start of each experiment, electrodes were lowered into the hippocampus, and depths were adjusted to maximize the amplitude of the negative-going dendritic fEPSPs elicited in CA1 by stimulation of CA3; typical depth profiles are shown in Fig. 6 (see Supplementary Methods for further information). Stimulation intensity was adjusted to elicit a contralateral fEPSP of ~3 mV in amplitude (200–500 μA). Representative fEPSPs evoked by stimulation of s1 i and s2 c are shown in Figs 1c and 6 . Table 1 shows mean stimulation intensities and baseline fEPSP slopes for all experiments, groups, and pathways. 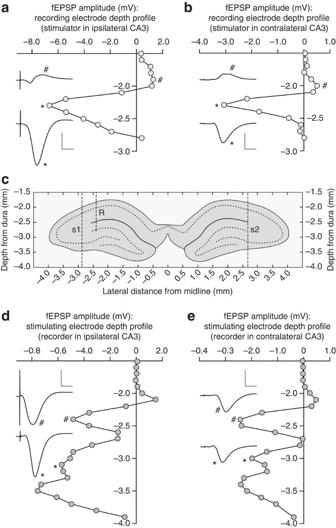Figure 6: Depth profiles during electrode implantation. (a,b) Changes in peak fEPSP amplitude elicited by ipsilateral (a) and contralateral (b). CA3 stimulation as a recording electrode is lowered into the hippocampus of a single rat; sample fEPSPs are shown at different depths (scale bar: vertical=3 mV; horizontal=5 ms); note the large negative-going responses elicited in the stratum radiatum by both ipsilateral and contralateral stimulation. (c) A schematic illustration of the locations of recording and stimulating electrode (see below) tracks in the same rat, based on the coronal section in which the location of the stimulating electrodes was most clearly visible. (d,e) Examples of fEPSP amplitude depth profiles recorded in the same animal as a stimulating electrode was lowered ipsilaterally (d) or contralaterally (e) relative to a stationary recording electrode in the stratum radiatum. Note the large negative-going responses elicited by both ipsilateral and contralateral stimulation of CA1 and CA3; sample fEPSPs are shown (scale bar: vertical=3 mV; horizontal=5 ms). See Supplementary Methods for more details. Figure 6: Depth profiles during electrode implantation. ( a , b ) Changes in peak fEPSP amplitude elicited by ipsilateral ( a ) and contralateral ( b ). CA3 stimulation as a recording electrode is lowered into the hippocampus of a single rat; sample fEPSPs are shown at different depths (scale bar: vertical=3 mV; horizontal=5 ms); note the large negative-going responses elicited in the stratum radiatum by both ipsilateral and contralateral stimulation. ( c ) A schematic illustration of the locations of recording and stimulating electrode (see below) tracks in the same rat, based on the coronal section in which the location of the stimulating electrodes was most clearly visible. ( d , e ) Examples of fEPSP amplitude depth profiles recorded in the same animal as a stimulating electrode was lowered ipsilaterally ( d ) or contralaterally ( e ) relative to a stationary recording electrode in the stratum radiatum. Note the large negative-going responses elicited by both ipsilateral and contralateral stimulation of CA1 and CA3; sample fEPSPs are shown (scale bar: vertical=3 mV; horizontal=5 ms). See Supplementary Methods for more details. Full size image The independence of s1 i and s2 c was confirmed at the start of the experiment in each animal by the delivery of pairs of biphasic stimulation pulses (50 μs per phase) to s2 c followed by s1 i at an interval of 50 ms (six pairs; 10-s intra-pair interval), followed by single test pulses delivered to s1 i only (6 pulses). PPF was calculated by expressing the mean fEPSP slope recorded in s1 i after stimulation of s2 c as a percentage of the value obtained in s1 i without prior stimulation. Mean data from all experiments reported in Figs 2 and 4 are shown in Fig. 1d (middle panel) and Table 1 . Paired stimulation was delivered first to s2 c , then to s1 i , as stimulation in the opposite sequence typically causes a modest paired-pulse depression of s2 c , a phenomenon that has been reported previously, and attributed to the recruitment of feed-forward and feedback inhibition by ipsilateral stimulation [59] . After electrode placement, and a check for the absence of PPF, baseline recording began; single biphasic test pulses (50-μs pulse width per phase) were delivered alternately to each stimulating electrode at 2-min intervals. The decision regarding the experiment to be conducted on any given day was always made before the start of baseline recording, with experiments alternating between groups across days. After a baseline period typically lasting several hours, and once stable fEPSPs had been observed for at least 1 h, tetanic stimulation began. Pulse width (per phase) was increased to 100 μs during a high-frequency tetanus. Strong tetanization consisted of three trains of 50 pulses at 250 Hz, with a 5-min inter-train interval; a weak tetanus comprised 1 train of 50 pulses at 100 Hz. Data obtained from a specific recording electrode were discounted if the fEPSP slope elicited by ipsilateral or bilateral stimulation fell to 60% of the baseline value or below within 4–5 h of tetanization (or the corresponding time point for untetanized pathways). In all cases, fEPSP slope data were normalized to the mean of the 1-h baseline period (assigned a value of 100%), and group means were calculated. Drugs An anisomycin solution was prepared by dissolving the powdered drug (Sigma-Aldrich, UK) in equimolar HCl and diluting with artificial cerebrospinal fluid (aCSF; in millimolar: 150 Na + , 3 K + , 1.4 Ca 2+ , 0.8 Mg 2+ , 155 Cl − , 0.2 H 2 PO 4 − , 0.8 HPO 4 2− , in pyrogen-free water at pH 7.2). The pH of the anisomycin solution was adjusted to 7.2 by the addition of NaOH, and the final concentration was 5 mg ml −1 . Powdered SCH23390 (Sigma-Aldrich, UK) was dissolved in sterile aCSF to yield a concentration of 5 mg ml −1 . Solutions were vortexed, gently sonicated and stored in small aliquots at −20 C before use. Drug administration and time lines In experiment 1, bilateral intraventricular (i.c.v.) infusion cannulae (24-gauge stainless steel) were lowered into the left and right lateral ventricles at the same time as electrode placement (co-ordinates: 0.9 mm posterior and 1.3 mm lateral to bregma; depth=−4.5 mm from the skull surface). Bilateral i.c.v. infusions (5 μl per ventricle over 10 min) were delivered via 5-μl SGE syringes mounted in a syringe pump (World Precision Instruments, Stevenage, UK), and connected to the infusion cannulae with plastic tubing. Control groups received a bilateral i.c.v. infusion (5 μl per ventricle over 10 min) of either anisomycin (5 μg μl −1 ) or aCSF starting 15 min before strong tetanization of s1 i . In the ‘rescue’ group, a strong tetanus was delivered to s2 c ending 15 min before infusion of anisomycin and subsequent strong tetanization of s1 i ; recording continued for a further 5 h. In experiment 2 ( Fig. 4 ), control groups received either strong or weak tetanization of s1 i in the absence of infusion; in the ‘rescue’ group, s1 i received weak tetanization 30 min before strong tetanization of s2 c ; recording continued for a further 5 h. In experiment 3, intra-hippocampal infusion cannulae were implanted under recoverable anaesthesia before electrophysiological recording. Rats were anaesthetized with isoflurane, injected with Rimadyl (carprofen; 5 mg kg −1 , s.c.), and placed in a stereotaxic frame with the skull horizontal. Guide cannulae (outer diameter=0.46 mm; Plastics One) were implanted bilaterally into the dorsal hippocampus (co-ordinates from bregma: AP=−4.5 mm; Lat.=3.0 mm; DV from dura=2.5 mm). These were fixed in place using dental cement, and the headcap was secured to the skull using jewellers’ screws. To prevent blockage or infection, dummy cannulae (or stylets; outer diameter=0.2 mm, protruding 0.5 mm from the end of the guide cannulae) were inserted into the guides during the recovery period. After ~1 week, the rats were anaesthetized with urethane for electrophysiological recording. After stable baseline recordings were obtained, injection needles were inserted into the guide cannulae. These were connected via plastic tubing to SGE syringes mounted in a syringe driver, and protruded 0.5 mm from the ends of the guide cannulae (that is, the infusion site was −3.0 mm from the dura). Intrahippocampal infusions of either aCSF or SCH23390 (5 μg μl −1 ; 1 μl per hippocampus) were delivered over 5 min, starting 15 min before strong tetanization of s1 i . Post-tetanus recording continued for 4 h in Experiment 3, rather than 5 h in Experiments 1 and 2. In order to control for infusion-induced baseline changes, after normalization with respect to baseline values (see above), fEPSP slopes in s1 i (tetanized pathway) were subsequently expressed as a percentage of the corresponding values in s2 c (control pathway) for each animal and time point. Histology At the end of experiments 1–3, marking lesions were made by the delivery of biphasic-mA constant-current pulses (1 s per phase) to both stimulating and recording electrodes. Rats were killed by cervical dislocation and brains were removed and stored in 10% formalin. Thirty-micrometre coronal sections through the hippocampus were then cut using a cryostat: 1 in 3 sections was mounted on a slide and stained with cresyl violet. After examination under a light microscope, stimulation sites were marked on the appropriate coronal section taken from the Paxinos and Watson atlas [60] . All electrodes were correctly positioned ( Fig. 7 and Supplementary Fig. S5 ), and, in experiment 1, all infusion cannulae were located in the lateral ventricles. 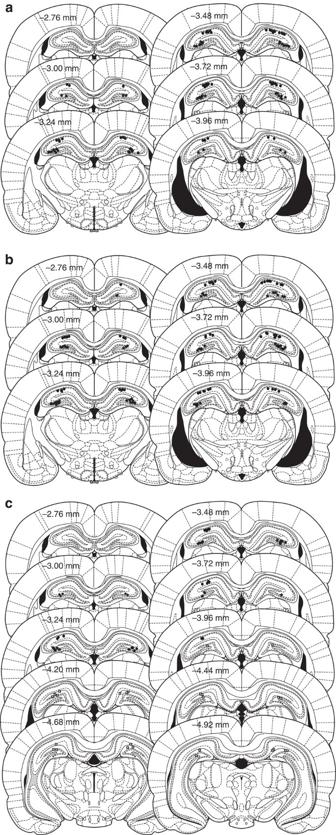Figure 7: Histology. Locations of the marking lesions made via all stimulating (filled stars) and recording electrodes (filled circles) used in Experiment 1 (a), Experiment 2 (b), and Experiment 3 (c); the locations of infusion cannulae are indicated by open squares in (c). Numbers indicate distance from bregma. Figures are adapted from Paxinos and Watson60. Figure 7: Histology. Locations of the marking lesions made via all stimulating (filled stars) and recording electrodes (filled circles) used in Experiment 1 ( a ), Experiment 2 ( b ), and Experiment 3 ( c ); the locations of infusion cannulae are indicated by open squares in ( c ). Numbers indicate distance from bregma. Figures are adapted from Paxinos and Watson [60] . Full size image How to cite this article: Shires, K.L. et al . Synaptic tagging and capture in the living rat. Nat. Commun. 3:1246 doi: 10.1038/ncomms2250 (2012).